Cell cycle-linked MeCP2 phosphorylation modulates adult neurogenesis involving the Notch signalling pathway Neuronal activity regulates the phosphorylation states at multiple sites on MeCP2 in postmitotic neurons. The precise control of the phosphorylation status of MeCP2 in neurons is critical for the normal development and function of the mammalian brain. However, it is unknown whether phosphorylation at any of the previously identified sites on MeCP2 can be induced by signals other than neuronal activity in other cell types, and what functions MeCP2 phosphorylation may have in those contexts. Here we show that in neural progenitor cells isolated from the adult mouse hippocampus, cell cycle-linked phosphorylation at serine 421 on MeCP2 is directly regulated by aurora kinase B and modulates the balance between proliferation and neural differentiation through the Notch signalling pathway. Our findings suggest MeCP2 S421 phosphorylation may function as a general epigenetic switch accessible by different extracellular stimuli through different signalling pathways for regulating diverse biological functions in different cell types. Methyl-CpG-binding protein 2 (MeCP2) is an important reader and interpreter of DNA methylation across the genome [1] . Mutations in MECP2 have been identified as the cause of Rett syndrome [2] , a severe neurodevelopmental disorder [3] . A better understanding of how extracellular signals access MeCP2 to generate adaptive functional outputs will provide valuable insights into how such a critical epigenetic interface influences normal and abnormal development and function of the mammalian nervous system. In postmitotic neurons, depolarization-induced Ca 2+ influx through voltage-gated calcium channels (VGCCs) has been shown to trigger phosphorylation of MeCP2 at serine 421 (S421) [4] , [5] , which is required for regulating synaptogenesis, dendritic morphology, synaptic scaling, long-term potentiation and spatial memory in the adult mouse brain [6] , [7] , [8] . To date, S421 phosphorylation has only been observed in postmitotic neurons [5] , [6] , [9] . Adult neurogenesis is a fascinating phenomenon that has attracted a lot of attention in recent years. Research in the field has mainly focused on the function of continued neurogenesis in adult life and the molecular mechanism underlying the process [10] , [11] . Evidence is just emerging to suggest a potential role of DNA methylation-dependent epigenetic mechanisms in regulating mammalian adult neurogenesis [12] , [13] , [14] , [15] . In this study we provide evidence that S421 is phosphorylated in adult neuroprogenitor cells (aNPC) isolated from the mouse hippocampus in response to growth signals. S421 phosphorylation in aNPC is linked to cell cycle and directly regulated by aurora kinase B, and plays a critical role in balancing aNPC proliferation/neural differentiation through the Notch signalling pathway. Our results suggest that in addition to the precise control of MeCP2 expression level, the regulation of posttranslational modification of MeCP2 is another mechanism underlying adult neurogenesis. In addition, stimulus-induced MeCP2 phosphorylation has the potential to function as a general epigenetic switch for regulating a diverse range of biological functions. Cell cycle-linked MeCP2 S421 phosphorylation in aNPCs We discovered that S421 was phosphorylated ( Fig. 1a ) in proliferating aNPCs isolated from the dentate gyrus (DG) of wild-type (WT) mouse hippocampus ( Supplementary Fig. 1a ). This phosphorylation was abolished in phosphor-mutant aNPCs isolated from the Mecp2 S421A;S424A/y hippocampus ( Fig. 1a ). Consistent with our previous report [6] , the level of total MeCP2 protein in aNPCs was indistinguishable between the WT and the phosphor mutant ( Fig. 1a,b ). When the WT aNPCs were differentiated into neurons, S421 phosphorylation first decreased, but then it increased again as the neurons matured ( Supplementary Fig. 1b ). As previous studies on postmitotic neurons have identified calcium influx through VGCCs as the trigger for S421 phosphorylation, we first tested whether they are involved in inducing S421 phosphorylation in aNPCs. Neither membrane depolarization by KCl nor treatment by Bay K8644, a calcium channel agonist, induced S421 phosphorylation in aNPCs ( Supplementary Fig. 1c ). Consistent with these results, Nimodipine, a VGCC blocker, failed to inhibit S421 phosphorylation in aNPCs ( Supplementary Fig. 1d,e ). In contrast, roscovitine, a broad-spectrum inhibitor of cyclin-dependent kinases (CDKs), significantly decreased S421 phosphorylation in aNPCs ( Supplementary Fig. 1d,e ). In light of this surprising result and the fact that aNPCs are dividing cells, we explored the possibility that growth factor and cell cycle regulation are involved in regulating S421 phosphorylation. Withdrawing growth factors led to concurrent decrease of phosphorylation of S421 ( Fig. 1c,d ) and the absence of G2/M phase cells ( Supplementary Fig. 2a ) in WT aNPCs. These alterations were unlikely to be secondary to potential cell fate changes, because expression of key cell-type markers remained similar before and after the withdrawal of growth factors ( Supplementary Fig. 2b,c ). To investigate whether S421 phosphorylation is linked to cell cycle, we arrested WT aNPCs at the G2/M phase with nocodazole ( Supplementary Fig. 2d,e ) or colchicine and observed a dramatic increase in the level of phospho-S421 ( Fig. 1e,f and Supplementary Fig. 2f ). Using a series of pharmacological reagents, we excluded the involvement of VGCCs, CaMKK and CaMKII in regulating cell cycle-linked S421 phosphorylation in aNPCs, because selective inhibitors of VGCCs, CaMKK or CaMKII failed to block cell cycle-linked S421 phosphorylation in these cells ( Supplementary Fig. 2g ). In contrast, roscovitine, a synthetic molecule with sub-μM IC50 values against CDK1, CDK2, CDK5, CDK7 and CDK9 (ref. 16 ), was highly effective in blocking nocodazole-induced S421 phosphorylation, suggesting that cell cycle-dependent kinases (CDKs) were upstream of S421 phosphorylation in aNPCs ( Fig. 1f,g ). As nocodazole and roscovitine together arrested slightly more cells at G1 than nocodazole alone ( Supplementary Fig. 2d,e ), roscovitine may have additional indirect effect on S421 phosphorylation through cell cycle alteration. Finally, such cell cycle-linked MeCP2 S421 phosphorylation was also observed in aNPCs isolated from the subventricular zone (SVZ) and NPCs isolated from neonatal brains ( Supplementary Fig. 2h ), raising the possibility that this may be a general phenomenon in proliferating cells. 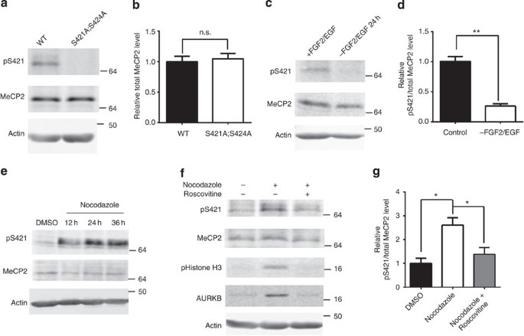Figure 1: Phosphorylation of MeCP2 S421 is regulated by cell cycle in aNPCs. (a,b) Western blot analysis of MeCP2 S421 phosphorylation and the quantification of total MeCP2 protein level in WT and phosphor-mutant aNPCs. (P=0.718, unpairedt-test with Welch’s correction,n=3 in each group). (c,d) Western blot analysis and quantification of the relative MeCP2 S421 phosphorylation level in WT aNPCs under normal proliferating condition and FGF-2/epidermal growth factor (EGF) withdrawal for 24 h. (n=3 in each group). (e) Western blot analysis reveals that MeCP2 S421 phosphorylation is induced by synchronizing aNPCs with nocodazole (150 ng ml−1). (f,g) Western blot analysis and quantification of the relative MeCP2 S421 phosphorylation level in aNPCs under conditions: (1) dimethyl sulphoxide (DMSO), (2) 36 h of nocodazole treatment, (3) 24 h of roscovitine (25 μM) treatment after pre-synchronization of the cells by nocodazole for 12 h. (n=3 in each group). Numbers next to western blottings are molecular weight markers. The bar graph shows the mean±s.e.m. *P<0.05, **P<0.01. Figure 1: Phosphorylation of MeCP2 S421 is regulated by cell cycle in aNPCs. ( a , b ) Western blot analysis of MeCP2 S421 phosphorylation and the quantification of total MeCP2 protein level in WT and phosphor-mutant aNPCs. ( P =0.718, unpaired t -test with Welch’s correction, n =3 in each group). ( c , d ) Western blot analysis and quantification of the relative MeCP2 S421 phosphorylation level in WT aNPCs under normal proliferating condition and FGF-2/epidermal growth factor (EGF) withdrawal for 24 h. ( n =3 in each group). ( e ) Western blot analysis reveals that MeCP2 S421 phosphorylation is induced by synchronizing aNPCs with nocodazole (150 ng ml −1 ). ( f , g ) Western blot analysis and quantification of the relative MeCP2 S421 phosphorylation level in aNPCs under conditions: (1) dimethyl sulphoxide (DMSO), (2) 36 h of nocodazole treatment, (3) 24 h of roscovitine (25 μM) treatment after pre-synchronization of the cells by nocodazole for 12 h. ( n =3 in each group). Numbers next to western blottings are molecular weight markers. The bar graph shows the mean±s.e.m. * P <0.05, ** P <0.01. Full size image Aurora kinase B directly phosphorylates MeCP2 S421 in aNPCs As the consensus sequence for the phosphorylation site of a CDK substrate, (serine/threonine)–proline–any amino acid–(lysine/arginine), is not found around S421, CDKs are unlikely to be the direct kinase for S421 in aNPCs. To search for the kinase that is directly responsible for phosphorylating S421 in aNPCs, we performed an in silico screen of consensus substrate sequences to identify a list of potential kinases, which was followed by a pharmacological screen in nocodazole-treated N2A cells. Aurora kinase B was the only candidate coming out of this two-step screen ( Supplementary Fig. 2i ). Consistent with previous reports that aurora kinase B is upregulated at the G2/M phase and downstream of CDKs [17] , [18] , we found that its level increased significantly in nocodazole-treated aNPCs, which was blocked by roscovitine ( Fig. 1f ). The phosphorylation level of serine 10 on histone 3, a known substrate of aurora kinase B [19] , closely followed the changes in the level of aurora kinase B in aNPCs ( Fig. 1f ). Hesperadin, a highly specific inhibitor of aurora kinase B, efficiently blocked cell cycle-linked S421 phosphorylation in aNPCs ( Fig. 2a,b and Supplementary Fig. 2j,k ), suggesting the aurora kinase B is required for S421 phosphorylation in these cells. To confirm this finding with an independent method, we generated lentivirus encoding short hairpin RNA (shRNA) specific for aurora kinase B ( Supplementary Fig. 2l ) and found it also significantly blocked cell cycle-linked S421 phosphorylation in aNPCs ( Fig. 2c,d ). As a negative control, a lentivirus encoding shRNA specific for enhanced green fluorescent protein (EGFP) had no effect on aurora kinase B level and S421 phosphorylation in aNPCs ( Fig. 2c,d ). To test whether MeCP2 and aurora kinase B physically interact with each other, we overexpressed epitope-tagged MeCP2 and aurora kinase B in Neuro2A cells and performed reciprocal co-immunoprecipitation followed by western blotting experiments. We found that flag-tagged aurora kinase B, but not flag-tagged EGFP, could pull down MeCP2 ( Fig. 2e ). Reversely, flag-tagged MeCP2, but not flag-tagged EGFP, could pull down aurora kinase B ( Fig. 2f ). Furthermore, the physical interaction between MeCP2 and aurora kinase B, as well as that between aurora kinase B and its known substrate, histone H3, can be detected in aNPCs arrested at the G2/M phase ( Fig. 2g ). Finally, when purified MeCP2 protein was incubated with aurora kinase B (but not an inactive form of the kinase-AURKB-DN) in the presence of ATP in an in vitro kinase assay, S421 was readily phosphorylated ( Fig. 2h ). Taken together, these results identify aurora kinase B as the direct kinase of MeCP2 S421 phosphorylation in aNPCs. 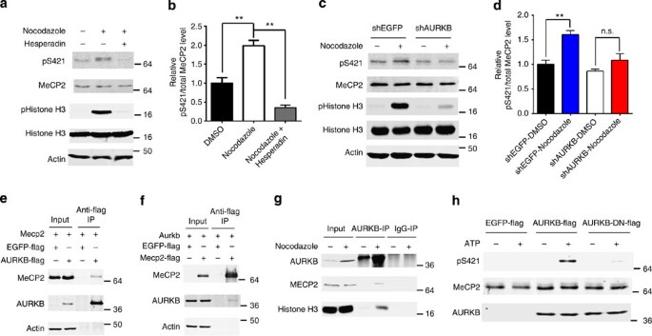Figure 2: Aurora kinase B is required for MeCP2 S421 phosphorylation in the aNPCs. (a,b) Western blot analysis and quantification of the relative MeCP2 S421 phosphorylation level in aNPCs: (1) dimethyl sulphoxide (DMSO), (2) 36 h of nocodazole (150 ng ml−1) treatment, (3) 24 h of hesperadin (2 μM) treatment after pre-synchronization of the cells by nocodazole for 12 h. (n=3 in each group). (c,d) Western blot analysis and quantification of the relative MeCP2 S421 phosphorylation level in EGFP-shRNA or AURKB-shRNA lentivirus-infected aNPCs, which are treated with DMSO or nocodazole for 24 h. (e,f) Western blot analysis reveals that MeCP2 and AURKB are co-immunoprecipitated reciprocally. (g) Western blot analysis reveals endogenous interaction between MeCP2 and AURKB in aNPCs. (h)In vitrokinase assay followed by western blotting demonstrates that AURKB can phosphorylate S421 on MeCP2. Numbers next to western blottings are molecular weight markers. Figure 2: Aurora kinase B is required for MeCP2 S421 phosphorylation in the aNPCs. ( a , b ) Western blot analysis and quantification of the relative MeCP2 S421 phosphorylation level in aNPCs: (1) dimethyl sulphoxide (DMSO), (2) 36 h of nocodazole (150 ng ml −1 ) treatment, (3) 24 h of hesperadin (2 μM) treatment after pre-synchronization of the cells by nocodazole for 12 h. ( n =3 in each group). ( c , d ) Western blot analysis and quantification of the relative MeCP2 S421 phosphorylation level in EGFP-shRNA or AURKB-shRNA lentivirus-infected aNPCs, which are treated with DMSO or nocodazole for 24 h. ( e , f ) Western blot analysis reveals that MeCP2 and AURKB are co-immunoprecipitated reciprocally. ( g ) Western blot analysis reveals endogenous interaction between MeCP2 and AURKB in aNPCs. ( h ) In vitro kinase assay followed by western blotting demonstrates that AURKB can phosphorylate S421 on MeCP2. Numbers next to western blottings are molecular weight markers. Full size image Altered proliferation/differentiation in phosphor-mutant NPC To reveal the functional significance of S421 phosphorylation in aNPCs, we examined proliferation and differentiation in both WT and phosphor-mutant aNPCs. Significantly fewer 5-bromo-2′-deoxyuridine (BrdU)-labelled Nestin + Sox2 + (triple positive) aNPCs were observed in phosphor-mutant compared with WT cells ( Fig. 3a,b and Supplementary Fig. 3a ), indicating a reduced proliferation potential. Although the phosphor-mutant aNPCs consistently took more time to grow than the WT aNPCs at each passage, no significant difference was found in the percentage of cells at each stages of the cell cycle ( Supplementary Fig. 3b ). On differentiation, significantly more Tuj1+ or MAP2+ positive cells were detected in phosphor-mutant compared with WT cells ( Fig. 3c,d and Supplementary Fig. 3c,d ), suggesting increased potential in neural differentiation. In contrast, no difference in glial differentiation was observed between the WT and phosphor-mutant aNPCs ( Fig. 3e,f ). Consistent with the stereological counting data ( Fig. 3c,f ), the messenger RNA levels of Tuj1 and NeuroD1 , two neuronal genes, were significantly higher in differentiated phosphor-mutant aNPCs than in WT aNPCs, while the mRNA levels of GFAP , a glial gene, remained unchanged in these cells ( Fig. 3g ). To validate our in vitro observations, we first performed BrdU labelling ( Fig. 3h,i ) to mark all the proliferating aNPCs in the subgranular zone of the hippocampus in adult mice and conducted unbiased stereological quantification throughout the DG of the hippocampus to compare the numbers of BrdU-labelled cells in the DG between Mecp2 S421A;S424A/y and WT littermates ( n =9 in each group). Fewer BrdU-labelled cells (89% of WT level) were found in the Mecp2 S421A;S424A/y hippocampus than in the WT littermate ( Fig. 3j , P =0.002, unpaired t -test with Welch’s correction). Consistent with the BrdU-labelling results, fewer Ki67 (a proliferation marker)-stained cells (65% of WT level) were found in the Mecp2 S421A;S424A/y hippocampus than in the WT littermates in stereological analysis an additional cohort of mice ( Fig. 3k , n =6 in each group, P =0.003, unpaired t -test with Welch’s correction). In addition to aNPC proliferation, we also examined the cell fates of these adult-born cells 4 weeks after they were born (as illustrated in Fig. 3l ). In the study, dividing aNPCs in the hippocampus of 8- to 9-week-old Mecp2 S421A;S424A/y mice ( n =9) and their WT littermates ( n =8) were first labelled by BrdU and given 4 weeks to differentiate. Sections throughout the hippocampus were triple labelled with an anti-BrdU antibody (to mark adult-born cells), an anti-NeuN antibody (to mark neurons) and an anti-S100β antibody (to mark glial cells). Under a confocal microscope, cells were identified as new neurons if they were positive for both BrdU and NeuN ( Fig. 3m , indicated by arrows), as new glial cells if they were positive for both BrdU and S100β ( Fig. 3m , indicated by an arrowhead), or as undetermined if they were only positive for BrdU. All BrdU-positive cells (407±132 in WT versus 379±81 in phosphor mutant, unpaired t -test with Welch’s correction, P =0.85) in the subgranular zone from all stained sections were included in the analysis. Our results showed that a higher proportion of the dividing aNPCs in the hippocampus of the Mecp2 S421A;S424A/y mice differentiated into neurons ( Fig. 3n , P =0.01, unpaired t -test with Welch’s correction) at the expense of undetermined cells ( Fig. 3n , P =0.02, unpaired t -test with Welch’s correction). As for the absolute number of BrdU-positive newborn neurons, no significant difference was detected between the Mecp2 S421A;S424A/y mice and their WT littermate (283±86 in WT versus 299±61 in phosphor mutant, unpaired t -test with Welch’s correction, P =0.88). The percentage of glial cells differentiated from the newborn cells in the adult hippocampus did not change significantly in the Mecp2 S421A;S424A/y mice when compared with the WT littermates ( Fig. 3n , P =0.48, unpaired t -test with Welch’s correction). No difference in the volume of granular cell layer was observed between the WT and phosphor-mutant mice ( Supplementary Fig. 3e ). Taken together, these in vitro and in vivo observations consistently identify a critical role of S421 phosphorylation in regulating aNPC proliferation and differentiation. 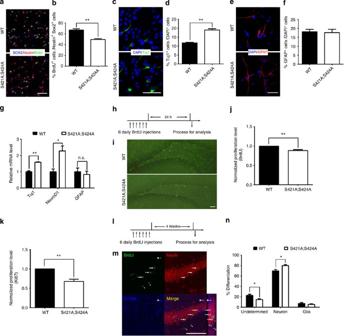Figure 3: Altered proliferation and differentiation of MeCP2 phosphor-mutant aNPCin vitroandin vivo. (a) Representative images of aNPCs isolated from WT andMecp2S421A;S424A/yhippocampus with BrdU pulse labelling, followed by immunocytochemistry analysis. (b) Quantification of the percentage of BrdU/Sox2/Nestin triple-labelled cells in WT andMecp2S421A;S424A/yaNPCs. (n=3 in each group). (c) Representative images of Tuj1+ neurons differentiated from WT andMecp2S421A;S424A/yaNPCs. (d) Quantification of the percentage of Tuj1+ cells in WT andMecp2S421A;S424A/yaNPCs on differentiation. (n=3 in each group). (e) Representative images of GFAP+ astrocyte differentiated from WT andMecp2S421A;S424A/yaNPCs. (f) Quantification of the percentage of GFAP+ cells in WT andMecp2S421A;S424A/yaNPCs on differentiation. (n=3 in each group). (g) Relative mRNA level of neuronal marker (Tuj1andNeuroD1) and astrocyte marker (GFAP) in WT andMecp2S421A;S424A/yaNPCs on differentiation, assayed by reverse transcriptase–qPCR. (n=3 in each group). (h) Schematics of the design of thein vivoBrdU labelling experiment. (i) Representative images of WT and theMecp2S421A;S424A/ybrain sections stained for BrdU immunoreactivity. (j) Quantification of relative number of BrdU+ cells obtained through stereological counting from WT andMecp2S421A;S424A/ymice (n=9 in each group). (k) Quantification of the relative number of Ki67+ cells obtained through stereological counting from WT andMecp2S421A;S424A/ymice (n=6 in each group). (l) Schematics of the design ofin vivoBrdU pulse/chase experiment to examine the differentiation profile of the adult-born hippocampal cells. (m) Representative confocal microscopy images to demonstrate how each cell type is identified. Three adult-born neurons (co-stained by BrdU and NeuN) are marked by arrow. One adult-born glial cell (co-stained by BrdU and S100b) is marked by arrowhead. Two adult-born undetermined cells (stained by BrdU only) are marked by asterisk. The rectangle panel to the right of the merged channel image is they–zview of the same optical stack. The optical size of thez-scan is 0.4 μm per step. (n) Quantification of proportions of the cell fate choices made by the dividing aNPCs in the hippocampus of WT andMecp2S421A;S424A/ymice. Scale bars, 50 μm. The bar graph shows the mean±s.e.m *P<0.05 **P<0.01. Figure 3: Altered proliferation and differentiation of MeCP2 phosphor-mutant aNPC in vitro and in vivo . ( a ) Representative images of aNPCs isolated from WT and Mecp2 S421A;S424A/y hippocampus with BrdU pulse labelling, followed by immunocytochemistry analysis. ( b ) Quantification of the percentage of BrdU/Sox2/Nestin triple-labelled cells in WT and Mecp2 S421A;S424A/y aNPCs. ( n =3 in each group). ( c ) Representative images of Tuj1+ neurons differentiated from WT and Mecp2 S421A;S424A/y aNPCs. ( d ) Quantification of the percentage of Tuj1+ cells in WT and Mecp2 S421A;S424A/y aNPCs on differentiation. ( n =3 in each group). ( e ) Representative images of GFAP+ astrocyte differentiated from WT and Mecp2 S421A;S424A/y aNPCs. ( f ) Quantification of the percentage of GFAP+ cells in WT and Mecp2 S421A;S424A/y aNPCs on differentiation. ( n =3 in each group). ( g ) Relative mRNA level of neuronal marker ( Tuj1 and NeuroD1 ) and astrocyte marker ( GFAP ) in WT and Mecp2 S421A;S424A/y aNPCs on differentiation, assayed by reverse transcriptase–qPCR. ( n =3 in each group). ( h ) Schematics of the design of the in vivo BrdU labelling experiment. ( i ) Representative images of WT and the Mecp2 S421A;S424A/y brain sections stained for BrdU immunoreactivity. ( j ) Quantification of relative number of BrdU+ cells obtained through stereological counting from WT and Mecp2 S421A;S424A/y mice ( n =9 in each group). ( k ) Quantification of the relative number of Ki67+ cells obtained through stereological counting from WT and Mecp2 S421A;S424A/y mice ( n =6 in each group). ( l ) Schematics of the design of in vivo BrdU pulse/chase experiment to examine the differentiation profile of the adult-born hippocampal cells. ( m ) Representative confocal microscopy images to demonstrate how each cell type is identified. Three adult-born neurons (co-stained by BrdU and NeuN) are marked by arrow. One adult-born glial cell (co-stained by BrdU and S100b) is marked by arrowhead. Two adult-born undetermined cells (stained by BrdU only) are marked by asterisk. The rectangle panel to the right of the merged channel image is the y–z view of the same optical stack. The optical size of the z -scan is 0.4 μm per step. ( n ) Quantification of proportions of the cell fate choices made by the dividing aNPCs in the hippocampus of WT and Mecp2 S421A;S424A/y mice. Scale bars, 50 μm. The bar graph shows the mean±s.e.m * P <0.05 ** P <0.01. Full size image Notch signalling is downstream of S421 phosphorylation in NPC To elucidate the molecular mechanism underlying the effect of S421 phosphorylation on balancing aNPC proliferation/neural differentiation, we performed transcription profiling in WT and phosphor-mutant aNPCs using the Neurogenesis and Neural Stem Cells PCR Array (Qiagen). Among the significant transcription changes in phosphor-mutant aNPCs, several belonged to the well-studied Notch signalling pathway ( Supplementary Fig. 4a ). Thus, we expanded our analysis to examine RNA levels of additional components of the Notch pathway, and found consistent decrease in the ligand ( Dll1 and Jag2 ), receptor ( Notch1 ) and several target genes ( Hes3 , Hes5 , Heyl and Hey1 ) of this pathway in phosphor-mutant aNPCs ( Fig. 4a,b and Supplementary Fig. 4b ). In addition, western blotting results confirmed the significant decrease in DLL1 protein level in phosphor-mutant aNPCs ( Fig. 4c,d ). As the link between ligand/receptor interaction on the cell membrane and target gene activation in the nucleus [20] , the intracellular domain of Notch (NICD) was found to be significantly lower in the phosphor-mutant aNPCs ( Fig. 4e,f ). Consistent with the idea that decreased Notch signalling in phosphor-mutant aNPC may underlie the observed changes in aNPC proliferation/differentiation, treatment of WT aNPCs with a Notch inhibitor led to decreased proliferation and increased neural differentiation similar to those observed in phosphor-mutant aNPCs ( Supplementary Fig. 4c,d ). Furthermore, we attempted to rescue the proliferation/differentiation phenotypes by overexpressing NICD in these cells. GFP- or NICD-expressing lentiviruses were produced and used to infect either WT or phosphor-mutant aNPCs. Although the NICD level in GFP-lentivirus-infected phosphor-mutant aNPCs remained much lower than that in GFP-lentivirus-infected WT aNPCs, the NICD level was similar between NICD-lentivirus-infected phosphor-mutant aNPCs and GFP-lentivirus-infected WT aNPCs ( Supplementary Fig. 4e ). In addition, overexpression of NICD, but not overexpression of GFP, was sufficient to reverse the reduced transcription of Notch signalling target genes in the phosphor-mutant aNPCs ( Fig. 4g ). Finally, the key phenotypes of reduced proliferation and increased neural differentiation in phosphor-mutant aNPCs were both rescued by the overexpression of NICD, as determined by comparing the number of BrdU-labelled aNPCs ( Fig. 4h,i ), the number of Tuj1-positive cells ( Fig. 4j,k ) and the expression level of Tuj1 and NeuroD1 RNA ( Fig. 4l ) on induction of differentiation in WT and phosphor-mutant aNPCs infected with either NICD or GFP lentiviruses. NICD expression did not lead to any significant change in glial differentiation in our aNPCs ( Supplementary Fig. 4f ). Interestingly, NICD overexpression in WT aNPCs did not alter either the cell cycle-linked S421 phosphorylation or the MeCP2 occupancy on the Notch1 promoter, further suggesting that Notch signalling is downstream of MeCP2 phosphorylation in aNPCs ( Supplementary Fig. 4g,h ). To distinguish the role of S421 phosphorylation regulation from that of overall MeCP2 expression regulation, we overexpressed MeCP2 in both the WT and phosphor-mutant aNPCs using a lentivirus encoding MeCP2. MeCP2 overexpression in WT aNPCs did not alter either Notch target gene transcription or the proliferation and neural differentiation of these cells ( Supplementary Fig. 4i–k ), nor did MeCP2 overexpression in the phosphor-mutant aNPCs rescue either the phenotype of decreased Notch target gene transcription or the phenotypes of decreased proliferation/increased neural differentiation in these cells ( Supplementary Fig. 4i–k ). Results from this series of experiments suggest that in this particular cell type, the epigenetic regulatory mechanism is at the level of phosphorylation but not the overall expression level of MeCP2. As the first step to reveal how MeCP2 phosphorylation may regulate Notch signalling, we conducted chromatin immunoprecipitation (ChIP) experiment to determine whether the phosphor-mutant MeCP2 protein has altered promoter occupancy at the promoters of Dll1 and Notch1 . We found increased binding of the phosphor-mutant protein at the promoters of both Dll1 and Notch1 ( Fig. 4m ), but not the promoter of Crh , a well-known MeCP2 target gene, or the major satellite repeats ( Supplementary Fig. 1 ). Similar promoter binding changes were observed when S421 phosphorylation was blocked by the aurora kinase B inhibitor hesperidin or by knocking down aurora kinase B ( Supplementary Fig. 4m,n ), suggesting aurora kinase B-regulated S421 phosphorylation may change MeCP2 binding to gene promoters. Together, these results indicate cell cycle-linked MeCP2 phosphorylation may directly regulate the transcription of both the ligand and receptor of Notch signalling pathway to influence aNPC proliferation and differentiation. 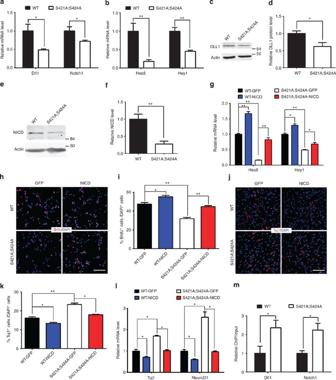Figure 4: Reduced Notch signalling in MeCP2 phosphor-mutant aNPCs and phenotypic rescue by NICD overexpression. (a) Reverse transcriptase (RT)–qPCR analysis of the relative mRNA level ofDll1andNotch1in WT andMecp2S421A;S424A/yaNPCs. (n=5 in each group forDll1,n=8 in each group forNotch1.) (b) RT–qPCR analysis of the relative mRNA level of Notch target geneHes5andHey1in WT andMecp2S421A;S424A/yaNPCs. (n=5 in each group.) (c,d) Western blot analysis and quantification of the relative protein level of DLL1 in WT andMecp2S421A;S424A/yaNPCs. (n=4 in each group.) (e,f) Western blot analysis and quantification of NICD level in WT andMecp2S421A;S424A/yaNPCs (n=5 in each group). (g) RT–qPCR analysis of the relative mRNA level ofHes5andHey1in WT andMecp2S421A;S424A/yaNPCs infected with GFP or NICD lentivirus. (n=3 in each group.) (h,i) Representative images and quantification of BrdU-labelled cells in WT andMecp2S421A;S424A/yaNPCs infected with GFP or NICD lentivirus, followed by BrdU pulse labelling. (n=3 in each group.) (j,k) Representative images and quantification of Tuj1+ neurons differentiated from WT andMecp2S421A;S424A/yaNPCs infected with GFP or NICD lentivirus. (n=3 in each group.) (l) Relative mRNA level of neuronal marker (Tuj1andNeuroD1) and astrocyte marker (GFAP) in WT andMecp2S421A;S424A/yaNPCs, which are infected with GFP or NICD lentivirus and then cultured in differentiation condition. (n=3 in each group.) Scale bar, 50 μm. (m) ChIP–qPCR analysis of the promoter occupancy of WT and phosphor-mutant MeCP2 onDll1andNotch1promoters. (n=4 in each group.) Numbers next to western blottings are molecular weight markers. The bar graphs in this figure show the mean±s.e.m. *P<0.05, **P<0.01. Figure 4: Reduced Notch signalling in MeCP2 phosphor-mutant aNPCs and phenotypic rescue by NICD overexpression. ( a ) Reverse transcriptase (RT)–qPCR analysis of the relative mRNA level of Dll1 and Notch1 in WT and Mecp2 S421A;S424A/y aNPCs. ( n =5 in each group for Dll1 , n =8 in each group for Notch1 .) ( b ) RT–qPCR analysis of the relative mRNA level of Notch target gene Hes5 and Hey1 in WT and Mecp2 S421A;S424A/y aNPCs. ( n =5 in each group.) ( c , d ) Western blot analysis and quantification of the relative protein level of DLL1 in WT and Mecp2 S421A;S424A/y aNPCs. ( n =4 in each group.) ( e , f ) Western blot analysis and quantification of NICD level in WT and Mecp2 S421A;S424A/y aNPCs ( n =5 in each group). ( g ) RT–qPCR analysis of the relative mRNA level of Hes5 and Hey1 in WT and Mecp2 S421A;S424A/y aNPCs infected with GFP or NICD lentivirus. ( n =3 in each group.) ( h , i ) Representative images and quantification of BrdU-labelled cells in WT and Mecp2 S421A;S424A/y aNPCs infected with GFP or NICD lentivirus, followed by BrdU pulse labelling. ( n =3 in each group.) ( j , k ) Representative images and quantification of Tuj1+ neurons differentiated from WT and Mecp2 S421A;S424A/y aNPCs infected with GFP or NICD lentivirus. ( n =3 in each group.) ( l ) Relative mRNA level of neuronal marker ( Tuj1 and NeuroD1 ) and astrocyte marker ( GFAP ) in WT and Mecp2 S421A;S424A/y aNPCs, which are infected with GFP or NICD lentivirus and then cultured in differentiation condition. ( n =3 in each group.) Scale bar, 50 μm. ( m ) ChIP–qPCR analysis of the promoter occupancy of WT and phosphor-mutant MeCP2 on Dll1 and Notch1 promoters. ( n =4 in each group.) Numbers next to western blottings are molecular weight markers. The bar graphs in this figure show the mean±s.e.m. * P <0.05, ** P <0.01. Full size image Three previous studies [12] , [13] , [14] have looked at the potential role of MeCP2 in regulating neurogenesis. Although these studies examined neurogenesis in three different spatial/temporal domains (adult hippocampus [12] , embryonic neural progenitors [14] and adult neural progenitors from the SVZ [13] ), all of them focused on the effect of overall expression level of MeCP2 on neurogenesis. In contrast, our current study highlights the phosphorylation, but not the overall expression level, of MeCP2 as a significant regulatory mechanism in regulating adult neurogenesis in the hippocampus. The complex signalling mechanism upstream of S421 phosphorylation suggests that MeCP2 phosphorylation is under precise control in aNPCs, which could be independent of the total level of MeCP2. Thus, it is not surprising that MeCP2 overexpression in aNPCs did not lead to any overt phenotypes in proliferation/differentiation. The fact that Smrt et al. [12] did not observe any significant change in aNPC proliferation/differentiation in the hippocampus of Mecp2 -null mice is not necessarily inconsistent with our findings in the Mecp2 phosphor-mutant mice, because other post-translational modifications on the MeCP2 protein may have opposing roles in regulating aNPC proliferation and differentiation. In WT cells, the two forces balance each other out. In S421A phosphor-mutant cells, the balance is lost and the phenotypes become evident. In Mecp2- null cells, the opposite regulatory roles of both S421 and the other uncharacterized modifications are lost. Thus, no overt aNPC proliferation/differentiation phenotypes could be observed. In addition to affecting neural differentiation, Tsujimura et al. [14] also observed changes in glial differentiation when MeCP2 is overexpressed in embryonic neural progenitors. The reason we did not observe similar changes in glial differentiation either in vitro or in vivo is probably due to the difference in developmental timing (adult versus embryonic) and the nature of MeCP2 changes (phosphorylation versus expression level). In comparing our findings with previous reports, another point worth noting is that the exact mechanism accessed by MeCP2 to regulate neurogenesis may be cell type specific. For instance, microRNAs, such as miR137, have been identified as the downstream effectors of MeCP2 in regulating the proliferation/differentiation of aNPCs isolated from the SVZ [13] . However, the level of miR137 expression is extremely low in our hippocampal aNPCs and is not significantly different between WT and Mecp2 phosphor mutant ( Supplementary Fig. 4o ). Therefore, although we cannot rule out a potential role of other microRNAs, miR137 expression is unlikely to be regulated by S421 phosphorylation and involved in regulating the proliferation/differentiation of hippocampal aNPCs. Moreover, given the wide distribution of MeCP2 across the genome [7] , [21] and many of the proteins it interacts to maintain normal cellular functions [22] , [23] , [24] , [25] , [26] , Notch signalling is unlikely to be the only misregulated pathway in the Mecp2 phosphor-mutant aNPCs. Future studies will be needed for a more complete understanding of the molecular events downstream of S421 phosphorylation in these cells. Finally, as both S421 and S424 were mutated in our study, it is a formal possibility that S424A also contributed to the phenotypes observed in the Mecp2 S421A;S424A/y aNPCs both in vitro and in vivo . Future studies on the Mecp2 S421A/y aNPCs and Mecp2 S421A/y mice are needed to evaluate this possibility. In summary, our study provides the first evidence that S421 of MeCP2 is phosphorylated in a proliferating cell type and plays a key role in regulating the proliferation and neural differentiation of aNPCs. Moreover, we have identified growth factors and CDKs as the signalling components upstream of S421 phosphorylation and aurora kinase B as the direct kinase for phosphorylating S421 in these cells. Finally, we have revealed Notch signalling as the molecular mechanism underlying the influence of S421 phosphorylation on the balance of proliferation and neural differentiation in these cells. Together with earlier studies on the regulation of S421 phosphorylation and its function in postmitotic neurons, our findings raise the possibility that S421 phosphorylation may function as a general regulatory switch accessible to diverse stimuli acting through distinct signalling pathways with important functional outcomes in different cell types. Animals All the experiments were performed using male mice. Mecp2 S421A;S424A/y mice have been backcrossed to C57BL/6 background for more than ten generations. Mice were housed in 12-h light (0600–1800, h)/12-h dark (1800–0600, h) cycle. Mice were housed <5 mice per cage. All protocols were approved by the Institutional Animal Care and Use Committee at University of Wisconsin–Madison. DNA construct The complementary DNAs of mouse Mecp2 , AurkB , the NICD and EGFP were subcloned to lentiviral expression vector. Sequence encoding the Flag peptide (DYKDDDDK) was introduced to the 3′-end of Mecp2 and AurkB cDNA by PCR. Expression of genes is driven by EF-1 Alpha (EF1α) promoter (pEF1α vector is a gift from Dr S.-c. Zhang’s lab). The mutation in AurkB-DN (dominant negative, K106R in the putative ATP-binding site) cDNA was generated by site-directed mutagenesis PCR. Lentiviral vector LentiLox 3.7 is used for expression of shRNA against EGFP and AurkB ( http://web.mit.edu/jacks-lab/protocols/pll37cloning.htm ). Sense and antisense target sequences of EGFP and AurkB were linked by loop sequence 5′-TTCAAGAGA-3′ and subcloned into LentiLox 3.7. Expression of shRNA is driven by U6 promoter. EGFP target sequence: 5′-gaacggcatcaaggtgaac-3′. AurkB target sequence: 5′-ggtaattcacagagacata-3′. Antibodies and drugs The following primary antibodies were used: Anti-MeCP2 (Cell Signaling, 3456, 1:2,000), Anti-MeCP2 (Abcam, ab50005, 1:2,000), Anti phospho-S421 (custom made by Covance, 1:2,000), anti-β-Actin (Sigma-Aldrich, a5441, 1:5,000), anti-AURKB (Millipore, 04-1036, 1:1,000; Cell Signalling, 3094, 1:1,000), anti-DLL1 (Abcam, Ab84620, 1:1,000), anti-NICD(Cell Signaling, 4147, 1:1,000), anti-phospho-Histone H3 (Ser10) (Cell Signalling, 3377, 1:1,000), anit-Histone H3 (Active Motif, 39163, 1:10,000), anti-S100b (SWANT, 1:500), anti-NeuN (Millipore, MAB377, 1:1,000), anti-BrdU (Accurate Chemical and Scientific, H7786, 1:1,000), anti-Ki67 (Dako, M7248, 1:500), anti-Tuj1 (Progema, G7121, 1:1,000), anti-MAP2 (Abcam, ab32454, 1:1,000), anti-GFAP (Dako, Z0334, 1:1,000), anti-Nestin (Aves labs, NES, 1:500), anti-SOX2 (Millipore, MAB4343, 1:1,000), anti-MCM2 (Santa Cruz, sc-9839, 1:1,000). DyLight 680/800-conjugated secondary antibodies (Thermo Fisher Scientific) were used for western blotting. Alexa Fluor-conjugated secondary antibodies (Invitrogen) were used for immunofluorescence staining. The following drugs were used: DAPT (Sigma-Aldrich), nocodazole (Sigma-Aldrich), colchicine (Sigma-Aldrich), roscovitine (Calbiochem), nimodipine (Sigma-Aldrich), Myr-CaMK IINtide (Calbiochem), STO-609 (Tocris), Bay K8644 (Calbiochem) and Hesperadin (Selleckchem). In vivo proliferation of NPCs in the adult hippocampus Tissue processing and in vivo cell proliferation analysis were performed as previously described [12] , [15] . Briefly, BrdU was dissolved in normal saline solution at a concentration of 10 mg ml −1 and filter sterilized. Eight- to nine-week-old mice received daily BrdU injections at the dose of 50 mg kg −1 body weight for 6 consecutive days, and were killed for analysis 24 h after the last (the sixth) BrdU injection. Stereological counting of the total number of BrdU or Ki67-labelled cells was performed under a Carl Zeiss Axioplan 2 Imaging microscope and the MBF Bioscience Stereo Investigator 8 software, using every sixth serial sections throughout the hippocampus. Scoring was performed without the knowledge of the genotype of the samples. In vivo differentiation of NPCs in the adult hippocampus Tissue processing and in vivo cell differentiation analysis were performed as previously described [12] , [15] . Briefly, BrdU was dissolved in normal saline solution at a concentration of 10 mg ml −1 and filter sterilized. Eight- to nine-week-old mice received daily BrdU injections at the dose of 50 mg kg −1 body weight for 6 consecutive days, and were killed for analysis 28 days after the last (the sixth) BrdU injection. Every sixth of the serial sections throughout the hippocampus were co-stained with an anti-BrdU antibody (to mark adult-born cells), an anti-NeuN antibody (to mark neurons) and an anti- S100β antibody (to mark glial cells). Quantification was done using a confocal microscope (Nikon Eclipse E600, with Nikon EZ-C1 3.50 software) to first look for immunoreactivity of BrdU, and then switch to the other channels to check whether a given BrdU-positive cell was also labelled by NeuN or S100β. Cells were identified as neurons if they were positive for both BrdU and NeuN, as glial cells if they were positive for both BrdU and S100β, or as undetermined if they were only positive for BrdU. All BrdU-positive cells in the subgranular zone from all stained sections were included in the analysis. Percentage of each cell fate in each mouse was determined by dividing the number of cells from each cell fate by the total number of BrdU-positive cells from the hippocampus of that mouse. Scoring was performed without the knowledge of the genotype of the samples. Immunohistochemistry Ten- to 12-week-old mice were transcardially perfused with normal saline solution followed by 4% paraformaldehyde (PFA). Brains were carefully dissected out, post-fixed in 4% PFA, cryoprotected in 30% sucrose, embedded and frozen in Tissue Tek. Serial coronal sections were cut at 40 μm throughout the brain and stained with appropriate primary and secondary antibodies. Isolation and culture of adult NPCs NPCs used in this study were isolated from the DG of 6- to 8-week-old male Mecp2 S421A;S424A mice and WT littermate controls based on published methods [27] . Briefly, DG was microdissected from 400 μm coronal sections of the forebrain. After enzymatic digestion using MACS Neural Tissue Dissociation kit (Miltenyi Biotech), DMEM/F-12 (Invitrogen) containing 10% FBS (Invitrogen) were added into each sample for stopping digestion. After filtering through a 70-μm cell strainer (BD Biosciences) and washing with DMEM/F-12, the single-cell suspension was collected and cultured with proliferation medium: Neurobasal medium (Invitrogen) containing 20 ng ml −1 basic fibroblast growth factor (FGF-2, Waisman Biomanufacturing), 20 ng ml −1 epidermal growth factor (Peprotech), B27 supplement (Invitrogen), Penicillin Streptomycin (Invitrogen) and L -glutamine (Invitrogen) in a 5% CO 2 incubator at 37 °C. Half of the medium was replaced every 2 days. Proliferation and differentiation assays of adult NPCs Proliferation and differentiation of aNPCs were analysed using published method [28] . Only early passage cells (between passage 4 and 10) and the same passage numbers of WT and Mecp2 S421A;S424A cells were used for the assay. For each experiment, stereological counting (Stereo Investigator, MBF Bioscience) of immunofluorescence-positive cells from duplicated wells were analysed and results were averaged as one data point ( n =1). At least three independent experiments ( n =3) were performed and used for statistical analyses for each analysis. In cell proliferation assay, we dissociated aNPCs with 0.05% Trypsin-EDTA (Invitrogen) for no longer than 1 min, stopped the digest with Trypsin inhibitor (Sigma-Aldrich) and finally plated the cells on poly- L -lysine/laminin-coated cover slips at a density of 100,000 cells per well in proliferation medium (see above). At 20 h post-plating, 5 μM BrdU (Sigma-Aldrich) was added into the culture medium for 8 h, after which the cells were fixed with 4% PFA for 30 min at room temperature. To detect BrdU incorporation, fixed cells were pretreated with 1 M HCl for 30 min at 37 °C and then washed with borate buffer, pH 8.5, for 30 min. We then followed our standard immunocytochemistry protocol. For the differentiation assay, aNPCs were treated similarly and plated as in the proliferation assay, but at a density of 50,000 cells per well. At 24 h post-plating, cells were changed into differentiation medium: Neurobasal medium with 1% B27 supplement, 1% Penicillin Streptomycin (Invitrogen), 2 mM L -glutamine(Invitrogen), 5 μM forskolin (Sigma-Aldrich), 1 μM retinoic acid (Sigma-Aldrich). Half of the medium was changed with fresh differentiation medium for 4 days, followed by fixation with 4% PFA for 30 min and standard immunocytochemistry protocol. Cell cycle analysis Cells were fixed in 2% PFA for 15 min at room temperature and stained with propidium iodide (50 μg ml −1 ) in the presence of RNase A (0.1 mg ml −1 ) for 40 min at 37 °C and then overnight at 4 °C. The stained cells were analysed on a FACS Calibur (BD Biosciences). Lentivirus preparation HEK293 cells were triple transfected using the calcium phosphate method with the lentiviral expression plasmid pEF1α-NICD, pEF1α-GFP, LentiLox 3.7-shEGFP or LentiLox 3.7-shAURKB and packaging vectors (pCAG-VSV-G and pCMVΔR8.91), and were switched to fresh media after 16 h. The supernatants containing the viral particles were collected 48 h after transfection and concentrated by ultracentrifuge (SW32 rotor, centrifuge at 25,000 r.p.m., 4 °C for 2.5 h). Transfection and co-immunoprecipitation Neuro2A cells (ATCC CCL-131) were maintained in DMEM (Invitrogen). Transfection of EGFP, Aurkb and Mecp2 expression plasmid was performed using Lipofectamine LTX with Plus Reagent (Invitrogen). For co-immunoprecipitation, transfected cells were lysed with cell lysis buffer (50 mM Tris-HCl, pH8.0, 170 mM NaCl, 0.5% NP-40, protease inhibitor (Roche), Phosphatase inhibitor (Sigma-Aldrich)), followed by sonication. Dynabeads (Invitrogen) were pre-washed with PBS/BSA (0.5% BSA in PBS) and incubated with antibody to form the beads/antibody complex. Protein lysis was then incubated with beads/antibody complex on a nutator at 4 °C overnight. The beads were washed three times with lysis buffer and finally boiled in Laemmli Sample Buffer (Bio-Rad) with 0.5% 2-Mercaptoethanol at 95 °C for 10 min. RNA extraction, and qRT–PCR and neural stem cell PCR array Total RNA was extracted from cultured adult NSCs using TRIzol Reagent (Invitrogen). The qScriptTM cDNA SuperMix kit (Quanta Biosciences) was used for cDNA synthesis. Real-time quantitative PCR (qPCR) was performed on StepOne Plus Real-Time PCR System (Applied Biosystems) using iQ SYBR Green Supermix (Bio-Rad). Fold change was calculated using the 2 −ΔCt method after normalization to Gapdh. For the sequences of all the qPCR primers used in this study, please see Supplementary Table 1 . For microRNA expression, a 15-μl reverse transcription reactions consisted of 5 ng of total RNA using TaqMan microRNA assay (mmu-miR-137 and snoRNA202) and Taqman MicroRNA Reverse Transcription Kit (Applied Biosystems) following the manufacturer’s recommendations. Real-time PCR was performed in StepOne Plus Real-Time PCR System using TaqMan microRNA assay (mmu-miR-137 and snoRNA202) and TaqMan Universal PCR Master Mix, No AmpErase UNG (Applied Biosystems) following the manufacturer’s recommendations. Relative level of miR-137 was calculated based on 2 −ΔCt method after normalization to the transcript level of snoRNA202 as the endogenous control. Neurogenesis and Neural Stem Cells PCR Array (Qiagen/SABiosciences, PAMM-404A, Version 3.0 system) was performed according to manufacturer’s instruction. Data were analysed using the online software from Qiagen/SABiosciences ( http://pcrdataanalysis.sabiosciences.com/pcr/arrayanalysis.php ). Western blot analysis Cultured adult NPCs were washed with PBS once and then lysed in Laemmli Sample Buffer (Bio-Rad) with 0.5% 2-Mercaptoethanol at 95 °C for 10 min. Sonication was used to lyse the cells and shear the genomic DNA, before the samples were subjected to SDS–PAGE. The protein samples were then transferred to Protran BA 85 nitrocellulose membranes (Whatman). The membrane was blocked by 5% dry milk and incubated with appropriate primary and DyLight dye-conjugated secondary antibodies. The Odyssey Western Detection Methods (LI-COR Biosciences) was used for signal detection. The integrated pixel intensity values for the target protein bands were analysed with NIH ImageJ software and then normalized to the intensity of the control β-Actin from the same samples. ChIP and gene-specific qPCR Cultured aNPCs were cross-linked with 1% formaldehyde for 15 min. Cross-linking was stopped by adding 1/20 volume of 2.5 M glycine. The following ChIP procedure was performed as previously described [6] . ChIP DNA and input DNA were dissolved in 20 μl of nuclease-free water and 1 μl of DNA was used for each real-time qPCR. Real-time qPCR was performed on StepOne Plus Real-Time PCR System (Applied Biosystems) using iQ SYBR Green Supermix (Bio-Rad). The ChIP DNA level was normalized to the input DNA level using the 2 −ΔCt method. Relative promoter occupancy was then calculated by setting the level of WT-MeCP2 binding as 1. Primers used in real-time PCR are: Dll1-ChIP: 5′-gtgttgagcatgccatgagc-3′ (forward), 5′-ctagctccaagaatcacacc-3′ (reverse) Notch1-ChIP: 5′-tataggcatcaggaggattg-3′ (forward), 5′-actcccttctacagaggctg-3′ (reverse) Crh-ChIP: 5′-gtcaccaaggaggcgataccta-3′ (forward), 5′-taaataatagggccctgccaag-3′ (reverse) Major Satellite-ChIP: 5′-catccacttgacgacttgaaaa-3′ (forward), 5′-gaggtccttcagtgtgcattt-3′ (reverse). Endogenous co-immunoprecipitation For co-immunoprecipitation, four 10-cm plates of confluently grown NPCs were lysed in cell lysis buffer (50 mM Tris-HCl, pH8.0, 170 mM NaCl, 0.5% NP-40, protease inhibitor (Roche), Phosphatase inhibitor (Sigma-Aldrich)), followed by sonication with a Bioruptor (Diagenode) for three 10-min periods. Cells were continuously lysed with rotation on a nutator at 4 °C for 30 min. Dynabeads (Invitrogen) were pre-washed with PBS/BSA (0.5% BSA in PBS) and incubated with antibody or IgG to form the beads/antibody complex. Protein lysate was then incubated with beads/antibody complex on a nutator at 4 °C overnight. The beads were washed three times with lysis buffer and finally boiled in Laemmli Sample Buffer (Bio-Rad) with 0.5% 2-Mercaptoethanol at 95 °C for 10 min. In vitro kinase assay Recombinant MeCP2 (0.5 μg; Prospec, PRO-212) was incubated with AURKB-flag, AURKB-DN-flag or EGFP-flag, which were freshly immunopurified from 293T cells, in Kinase buffer (50 mM HEPES, pH 7.5, 150 mM NaCl, 10 mM MgCl 2 , 1 mM dithiothreitol, protease inhibitor (Roche), Phosphatase inhibitor (Sigma-Aldrich)) with or without 100 μM ATP at 30 °C for 30 min. The presence of phosphorylated S421 was detected by western blotting with anti-phospho-S421 antibody. Statistical analysis No statistical methods were used to predetermine sample sizes, but the samples sizes we used were consistent with those generally employed in the field. Data were first tested for normality using the D'Agostino-Pearson omnibus test when necessary. Comparisons between two groups were analysed by unpaired t -test with Welch’s correction. Multiple comparisons in the same data set were analysed by one-way analysis of variance followed by Tukey’s multiple comparisons test. Data from multiple groups with multiple treatments were analysed by two-way analysis of variance followed by Tukey’s multiple comparisons test. P <0.05 was considered to be statistically significant. Statistical processing was performed using Microsoft Excel and GraphPad Prism Software. How to cite this article: Li, H. et al. Cell cycle-linked MeCP2 phosphorylation modulates adult neurogenesis involving the Notch signalling pathway. Nat. Commun. 5:5601 doi: 10.1038/ncomms6601 (2014).